Reactive oxygen species mediate pollen tube rupture to release sperm for fertilization inArabidopsis In flowering plants, sperm are transported inside pollen tubes to the female gametophyte for fertilization. The female gametophyte induces rupture of the penetrating pollen tube, resulting in sperm release and rendering them available for fertilization. Here we utilize the Arabidopsis FERONIA (FER) receptor kinase mutants, whose female gametophytes fail to induce pollen tube rupture, to decipher the molecular mechanism of this critical male–female interactive step. We show that FER controls the production of high levels of reactive oxygen species at the entrance to the female gametophyte to induce pollen tube rupture and sperm release. Pollen tube growth assays in vitro and in the pistil demonstrate that hydroxyl free radicals are likely the most reactive oxygen molecules, and they induce pollen tube rupture in a Ca 2+ -dependent process involving Ca 2+ channel activation. Our results provide evidence for a RHO GTPase-based signalling mechanism to mediate sperm release for fertilization in plants. Unlike fertilization in animal where flagellated sperm swim to fuse with the oocyte, sperm cells in flowering plants are immotile. They are borne inside the pollen tube, the male gametophyte, and rely on its polarized growth inside the female organ, pistil, for transportation and delivery to the female gametophyte located inside an ovule for fertilization ( Fig. 1a ) [1] , [2] , [3] . The egg cell and a pair of synergid cells are located at one end of the female gametophyte, close to the ovular aperture called micropyle. Pollen tube growth in the pistil is highly regulated and fertilization is achieved only after a series of interactive events between the penetrating pollen tube and specific pistil tissues [4] , [5] , [6] and cells [7] , [8] . Guided by female cues [7] , [8] , the pollen tube enters the ovule via the micropyle. The filiform apparatus is located at the entrance of the female gametophyte. It is a thickened cell wall region crisscrossed by an abundance of cell membrane protrusions from the synergids [9] , [10] , the pair of cells flanking the egg ( Fig. 1a ). The pollen tube invades one of the synergids whereupon it ruptures, ejecting sperm and rendering them available for fertilization [3] , [11] . Late-arriving pollen tubes are repelled from entering an already penetrated ovule. 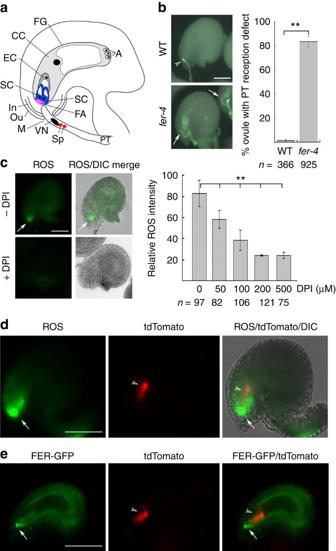Figure 1: FER mediates a ROS maximum at the filiform apparatus/synergid cell region. (a) An ovule sketch showing a penetrating pollen tube. A, antipodal cells; FG, female gametohyte; CC, central cell; EC, egg cell; SC, synergid cell; FA, filiform apparatus; In, Oi, inner and outer integuments; M, micropyle; PT, pollen tube; VN, pollen tube vegetative nucleus; Sp, sperm cell. (b) Aniline blue-stained WT andfer-4ovules (left) and quantification of pollen tube (PT)–ovule interaction defects (right). Arrowhead, a single, ruptured tube; arrows, multiple overgrown (reflecting non-rupture) tubes appearing as thick bundles. Data=average±s.e.m. from at least triplicate samples (each with at least three pistils) from a representative analysis;n=total number of ovules examined. **P≤0.01 by Student’st-test. (c) H2DCF-DA staining to show ovular ROS (left panel) and dose-dependent DPI inhibition (right panel). For comparative ROS analysis, a region of interest (ROI) with identical areas at the synergid cell/filiform apparatus region (Supplementary Fig. 2) from the ovules compared was quantified by ImageJ. Data in histogram=average±s.d. of ovules from at least three pistils (n=number of ovules examined) from a representative of three independent analyses. (d,e) Co-imaging of the discharged pollen tube cytoplasm (red, arrowheads) and ROS (green, arrows) in a wild-type ovule (d) and of pollen tube cytoplasm (red, arrowheads) and with FER-GFP (green, arrows) in apFER::FER-GFPtransformed ovule (e). Figure 1: FER mediates a ROS maximum at the filiform apparatus/synergid cell region. ( a ) An ovule sketch showing a penetrating pollen tube. A, antipodal cells; FG, female gametohyte; CC, central cell; EC, egg cell; SC, synergid cell; FA, filiform apparatus; In, Oi, inner and outer integuments; M, micropyle; PT, pollen tube; VN, pollen tube vegetative nucleus; Sp, sperm cell. ( b ) Aniline blue-stained WT and fer-4 ovules (left) and quantification of pollen tube (PT)–ovule interaction defects (right). Arrowhead, a single, ruptured tube; arrows, multiple overgrown (reflecting non-rupture) tubes appearing as thick bundles. Data=average±s.e.m. from at least triplicate samples (each with at least three pistils) from a representative analysis; n =total number of ovules examined. ** P ≤0.01 by Student’s t -test. ( c ) H 2 DCF-DA staining to show ovular ROS (left panel) and dose-dependent DPI inhibition (right panel). For comparative ROS analysis, a region of interest (ROI) with identical areas at the synergid cell/filiform apparatus region ( Supplementary Fig. 2 ) from the ovules compared was quantified by ImageJ. Data in histogram=average±s.d. of ovules from at least three pistils ( n =number of ovules examined) from a representative of three independent analyses. ( d , e ) Co-imaging of the discharged pollen tube cytoplasm (red, arrowheads) and ROS (green, arrows) in a wild-type ovule ( d ) and of pollen tube cytoplasm (red, arrowheads) and with FER-GFP (green, arrows) in a pFER :: FER-GFP transformed ovule ( e ). Full size image Mutant analyses showed that the female gametophyte plays a determining role in inducing sperm release and preventing late-arriving tubes from entering an already penetrated ovule [12] , [13] , [14] , [15] , [16] , [17] while the male gametophyte is also actively involved to ensure reproductive success [18] , [19] , [20] , [21] . Among these mutants, ovules in loss-of-function mutants in the Arabidopsis FERONIA/SIRÈNE receptor kinase (FER/SRN, FER is used from here on except when referring to the srn mutant) show the strongest dual phenotype of failing to induce pollen tube rupture and preventing multiple tube entrance. As a consequence, fer ovules exhibit a readily notable phenotype of pollen tube pile up ( Supplementary Fig. 1a ) due to overgrowth of one or more pollen tubes inside the female gametophyte [12] , [13] . FER is a member of the Arabidopsis THESEUS1/FER receptor-like kinase (RLK) family [22] ; the functions of THESEUS1, which regulates growth in cellulose-deficient seedlings, and FER are the first in the family to be elucidated [23] , [24] . FER is broadly expressed [24] , [25] , except in the pollen [26] , where several related RLKs are expressed [26] , [27] , [28] . Two of these pollen-specific RLKs, ANXUR1 and ANXUR2, function redundantly to ensure pollen tube integrity [27] , [28] . Double anxur1/2 mutants show precocious pollen tube rupture in the pistil, never reaching the ovules for fertilization. FER is also important for overall growth and development, regulating cell growth, hormone-signalled responses [25] , [29] , [30] , [31] , and facilitates pathogen invasion [16] . We showed previously [25] that FER interacts with ROPGEFs [32] , guanine nucleotide exchange factors that activate RAC/ROP GTPases (plant RHOs) and major molecular switches that mediate myriad signal-response systems [33] , [34] , [35] . We showed that FER functions as a cell surface regulator in a FER-ROPGEF-RAC/ROP complex to stimulate nicotinamide adenine dinucleotide phosphate (NADPH) oxidase-produced reactive oxygen species (ROS) in roots and mediate polarized root hair growth [25] . Since FER interacts with multiple ROPGEFs, which are known to interact with distinct classes of effectors [36] , [37] , whether FER uses the same or other RAC/ROP-regulated pathways to mediate its various functional roles has to be established on a case by case basis. On the other hand, despite the accumulating knowledge on the genetic control over male–female gametophyte interactions [3] , [11] , insights pertaining to the mechanisms that underlie these processes remain sparse due to the difficulty to access and manipulate the microenvironment for the male–female encounter. Thus far, only a female gametophyte produced defensin-like protein, ZmES4, from maize has been shown to burst pollen tubes, acting preferentially on maize pollen tubes [17] . Therefore, discovery of a FER to ROS signalling pathway operating in roots [25] provided a valuable portal to explore how the female gametophyte controls the fate of the invading male gametophyte. Here we show that FER induces a high ROS environment at the entrance of the female gametophyte and that it is required for inducing pollen tube rupture. In particular, we show that inhibiting female gametophytic ROS production phenocopies the fer ovule phenotype of pollen tube overgrowth and provide evidence for ROS-induced pollen tube rupture as a Ca 2+ -dependent process in vitro and in the pistil. Our results establish a model whereby FER interacts with the RAC/ROP molecular switch and acts via a NADPH oxidase-dependent signalling pathway to induce sperm release and enable fertilization in flowering plants. FER mediates high ROS levels at the filiform apparatus area As the FER-regulated reproductive phenotype was originally described in heterozygous srn [12] and fer [13] mutants and our study would be carried out in the homozygous T-DNA induced fer-4 null mutant [25] , we first ascertained that fer-4 has a reproductive phenotype indistingusishable from those reported in srn and fer . We established that pollen tubes failed to rupture in about 80% of the fer-4 ovules and that about half of these were also penetrated by multiple pollen tubes ( Fig. 1b ; Supplementary Fig. 1a,b ), levels that approximately doubled those reported in heterozygous srn- and fer- mutant pistils. We also confirmed that reduced fertility in fer-4 was female dependent ( Supplementary Fig. 1c,d ), just as previously reported for the heterozygous srn and fer . To examine whether female gametophyte-expressed FER [24] ( Supplementary Fig. 2 ) regulates ROS production, wild-type ovules were stained for ROS in the absence and presence of diphenyl iodonium chloride (DPI), an inhibitor commonly used to assess cell membrane NADPH oxidase-dependent ROS synthesis ( Supplementary Fig. 3 ) [25] , [38] , [39] . Results showed a DPI-sensitive ROS maximum at the filiform apparatus/synergid cell region ( Fig. 1c ; Supplementary Fig. 2 ), where FER is prominently located [24] ( Supplementary Fig. 2 ). We also co-imaged red fluorescent cytoplasm discharged from ruptured tdTomato-expressing pollen tubes in the synergid cell with ROS in wild-type ovules ( Fig. 1d ) or with FER-GFP in ovules from FER promoter ( pFER) :: FER-GFP transformed plants [25] ( Fig. 1e ). Results showed a close spatial relationship between FER and ROS at the entrance to the female gametophyte, just external to the red fluorescence-labelled pollen tube cytoplasm. We then examined the ROS status and FER expression during floral development [40] , [41] ( Supplementary Fig. 4a ) and compared the ROS status between wild type and fer -mutant ovules. pFER -expressed FER-GFP and ROS both showed a developmentally regulated accumulation pattern in wild-type ovules, peaking during floral stages 13–15 ( Fig. 2a ) when ovules were at their prime receptivity for pollen tubes [40] , [41] (See Supplementary Fig. 4a ), and dropping by stage 16 when fertilization was complete. On the other hand, ROS level remained low in fer-4 throughout development ( Fig. 2b,c ; Supplementary Fig. 4b,c ). The female gametophytic ROS status in srn showed a similar developmental regulation profile ( Fig. 2d ), further ascertaining that loss of a high ROS environment at the entrance to the female gametopyte has resulted from loss of FER function. Taken together, these observations are consistent with FER mediating a NADPH oxidase-dependent ROS maximum at the filiform apparatus/synergid cell region of the female gametophyte and that ROS potentially play a role in the FER-regulated reproductive processes. 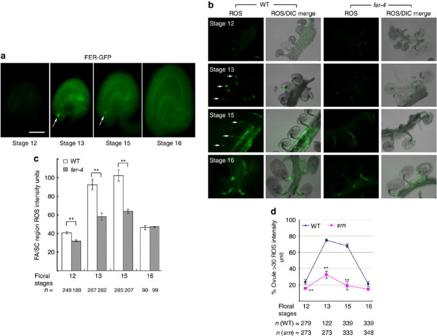Figure 2: FER mediates a developmentally regulated ROS maximum at the entrance to the female gametophyte. (a)pFER::FER-GFPexpression in floral developmental stages 12–16 (refs40,41). Arrows indicate filiform apparatus/synergid cell region. (b) H2DCF-DA-stained wild-type andfer-4ovular ROS. Arrows indicate micropylar regions. (c,d) Quantitative analysis of H2DCF-DA-detected female gametophytic ROS in wild-type andfer-4(c) and in wild-type andsrn(d) ovules. (c) compares average filiform apparatus/synergid cell (FA/SC) region ROS intensity units; (d) compares % of ovules with ROS intensity above the baseline threshold set at 30 ROS intensity units. Both methods, and a third, comparing the ratio between FA/SC ROS and chalazal end ROS (around the antipodal cells), and comparisons using a second ROS-stain, HPF38,69(Supplementary Fig. 4b,c), yielded comparable results. Quantitative data (c,d) are averages±s.e.m. of triplicate samplings (each with at least three pistils) from an analysis representative of three independent experiments; **, significant differences,P<0.01 by Student’st-test.n=total number of ovules examined. Scale bar, 50 μm. Figure 2: FER mediates a developmentally regulated ROS maximum at the entrance to the female gametophyte. ( a ) pFER::FER-GFP expression in floral developmental stages 12–16 (refs 40 , 41 ). Arrows indicate filiform apparatus/synergid cell region. ( b ) H 2 DCF-DA-stained wild-type and fer-4 ovular ROS. Arrows indicate micropylar regions. ( c , d ) Quantitative analysis of H 2 DCF-DA-detected female gametophytic ROS in wild-type and fer-4 ( c ) and in wild-type and srn ( d ) ovules. ( c ) compares average filiform apparatus/synergid cell (FA/SC) region ROS intensity units; ( d ) compares % of ovules with ROS intensity above the baseline threshold set at 30 ROS intensity units. Both methods, and a third, comparing the ratio between FA/SC ROS and chalazal end ROS (around the antipodal cells), and comparisons using a second ROS-stain, HPF [38] , [69] ( Supplementary Fig. 4b,c ), yielded comparable results. Quantitative data ( c , d ) are averages±s.e.m. of triplicate samplings (each with at least three pistils) from an analysis representative of three independent experiments; **, significant differences, P <0.01 by Student’s t -test. n =total number of ovules examined. Scale bar, 50 μm. Full size image Female gametophytic ROS are required for pollen tube rupture Lacking genetic suppressors for fer mutants that were originally reported in 2003 (refs 12 , 13 ), and without a loss-of-function NADPH oxidase mutant that does not severely impair growth and development rendering precise interpretation of reproductive anomalies difficult, we devised a pistil-feeding assay to manipulate the pistillate environment ( Fig. 3a ; Supplementary Fig. 5a,b ) to determine whether ROS indeed underlie FER-regulated pollen tube–ovule interactions. Feeding wild-type pistils with DPI effectively suppressed ovule ROS ( Supplementary Fig. 5c,d ) and pollen tube rupture, resulting in their overgrowth ( Fig. 3b,c , white bars). Similarly, scavenging superoxide and hydroxyl radical (see Supplementary Fig. 3 ) reduced ovule ROS and prevented pollen tube rupture ( Fig. 3d,e ; Supplementary Fig. 5e ). Together, these observations provide strong support for ROS being required for pollen tube rupture in the female gametophyte. On the other hand and unlike the dual phenotype of pollen tube overgrowth and supernumerary pollen tube entrance in fer ovules, obliterating female gametophytic ROS and preventing pollen tube rupture had no impact on the wild-type ovule ability to prevent multiple tube entrance ( Fig. 3b,c , grey bars). These results show that although intimately linked, the two FER-regulated pollen tube–ovule interactive processes can be uncoupled. 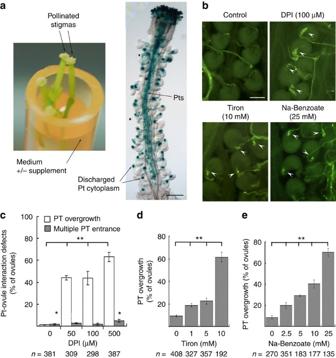Figure 3: ROS induce pollen tube rupture in the female gametophytes. (a) Pistil-feeding assay. Excised wild-type pistils maintained in a reservoir of feeding medium and a single wild-type pistil pollinated by GUS-expressing pollen highlighting ovule targeting and cytoplasmic discharge (blue dots) in the female gametophytes.Supplementary Figure 5ashows an aniline blue-stained pollinated pistil after growth in the pistil-feeding assay, also confirming that normal pollen tube growth and ovule targeting were not affected. Whenfer-4pistils were maintained in the pistil-feeding assays, they retained pollen tube–ovule interaction defects, harbouring comparable levels of pollen tube overgrowth as seen in pistils pollinatedin planta(Supplementary Fig. 5b), confirming that the FER-regulated process was not affected in these assays. (b–e) Pollen tube rupture and entrance property in ovules from mock-treated (control) wild-type pistils and those fed with DPI, tiron and Na-benzoate. DPI inhibition is commonly used as a reflection of NADPH oxidase-dependent ROS synthesis, tiron and Na-benzoate are commonly used ROS scavengers67(Supplementary Fig. 3). Arrowheads in (b) indicate overgrown single-pollen tubes. ROS levels were reduced to almost non-detectable level in these treated ovules (Supplementary Fig. 5c,d). CuCl2, another ROS scavenger (Supplementary Fig. 3), also reduced ovular ROS and induced pollen tube overgrowth (Supplementary Fig. 5d,e). Data=average ±s.e.m. from at least triplicate samples (each with at least three pistils) representative of three independent experiments;n=total number of ovules examined. **P≤0.01; *P≤0.05 as determined by Student’st-tests. Scale bars, 250 μm (a); 100 μm (b). Figure 3: ROS induce pollen tube rupture in the female gametophytes. ( a ) Pistil-feeding assay. Excised wild-type pistils maintained in a reservoir of feeding medium and a single wild-type pistil pollinated by GUS-expressing pollen highlighting ovule targeting and cytoplasmic discharge (blue dots) in the female gametophytes. Supplementary Figure 5a shows an aniline blue-stained pollinated pistil after growth in the pistil-feeding assay, also confirming that normal pollen tube growth and ovule targeting were not affected. 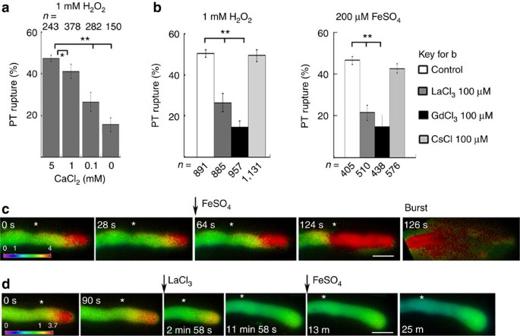Figure 5: ROS-induced pollen tube rupture is Ca2+dependent. (a) Effect of reducing [Ca2+] on H2O2-induced pollen tube rupture. The excised pistils were pollinated and initially maintained in solidified medium containing 100 μM Ca2+to allow germination and tube growth prior to application of liquid medium containing 5 mM (standard) to 0 Ca2+. The level of tube rupture under 0 Ca2+treatment condition reflected the presence of minuscule amount of residual Ca2+contributed from the original growth medium. (b) Effects of inhibitors of Ca2+channel (LaCl3, GdCl3) and K+channel (CsCl) on ROS-induced rupture. Pollen tube rupture was suppressed by LaCl3and GdCl3in a dose-dependent manner but was insensitive to CsCl and control reagents MgCl2and BaCl217(Supplementary Fig. 7a–d). (c,d) Imaging intracellular Ca2+in a Ca2+-sensitive cameleon-expressing pollen tube during ROS (250 μM FeSO4)-induced rupture (c) and in the presence of 100 μM LaCl3(d). Heat maps reflect relative Ca2+levels. The 0 s images show high Ca2+at the tube apical region, typical of elongating pollen tubes1,42. * indicate the same position on the pollen tubes as reference points for growth during the observation period. LaCl3-treated tube continued growth during the treatment period (see distance between * and tip), slowed and developed apical swelling (d), but did not burst.Supplementary Movies 3 and 4show the time series in (c). Scale bar, 10 μm. Data (a,b)=average±s.e.m. from at least triplicate samples representative of three independent experiments;n=total number of pollen tubes examined. **P≤0.01 by Student’st-tests. When fer-4 pistils were maintained in the pistil-feeding assays, they retained pollen tube–ovule interaction defects, harbouring comparable levels of pollen tube overgrowth as seen in pistils pollinated in planta ( Supplementary Fig. 5b ), confirming that the FER-regulated process was not affected in these assays. ( b – e ) Pollen tube rupture and entrance property in ovules from mock-treated (control) wild-type pistils and those fed with DPI, tiron and Na-benzoate. DPI inhibition is commonly used as a reflection of NADPH oxidase-dependent ROS synthesis, tiron and Na-benzoate are commonly used ROS scavengers [67] ( Supplementary Fig. 3 ). Arrowheads in ( b ) indicate overgrown single-pollen tubes. ROS levels were reduced to almost non-detectable level in these treated ovules ( Supplementary Fig. 5c,d ). CuCl 2 , another ROS scavenger ( Supplementary Fig. 3 ), also reduced ovular ROS and induced pollen tube overgrowth ( Supplementary Fig. 5d,e ). Data=average ±s.e.m. from at least triplicate samples (each with at least three pistils) representative of three independent experiments; n =total number of ovules examined. ** P ≤0.01; * P ≤0.05 as determined by Student’s t -tests. Scale bars, 250 μm ( a ); 100 μm ( b ). Full size image ROS induce pollen tube rupture in vitro To further decipher the mechanism behind the ROS-induced pollen tube rupture process, we used the semi- in vivo pollen tube growth system [4] , [42] to explore how pollen tubes would respond to applied ROS. Arabidopsis pollen tubes emerging from pollinated pistils cultured on standard growth medium showed robust growth for at least 4–6 h ( Fig. 4a ). To generate a high ROS condition, we added xanthine/xanthine oxidase (X/XO) to convert molecular oxygen to superoxide, or applied H 2 O 2 directly, or used FeSO 4 to generate hydroxyl radicals via the Fenton reaction [38] , [43] , [44] ( Supplementary Fig. 3 ). All of these applications caused an abrupt and explosive discharge of pollen tube cytoplasm and sperm cells ( Fig. 4a–c ; Supplementary Fig. 6a–d ; Supplementary Movies 1,2). Hydroxyl radical scavengers effectively suppressed rupture induced by all three reagents ( Fig. 4d–f ; Supplementary Fig. 6e–g ). These observations imply that the X/XO-generated superoxide and the directly added H 2 O 2 had predominantly acted via their conversion into hydroxyl radicals. Taken together, with observations from pistil-feeding assays ( Fig. 3 ; Supplementary Fig. 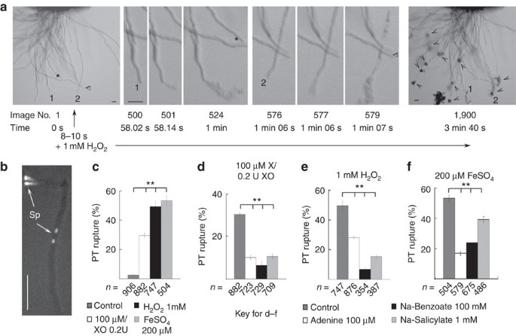5 ), these results also implicate hydroxyl radicals as the most prevalent active oxygen species that induce pollen tube rupture in the female gametophyte. Figure 4: ROS induce pollen tube rupturein vitro. (a) H2O2-induced tube rupture. The entire sample immediately prior to application of ROS (0 s) and when a majority of the pollen tubes has ruptured (3 m 40 s) (arrowheads point to cytoplasmic discharges) is shown in full. Magnified views of the first two rupturing pollen tubes (1, 2) are shown in between. * and Δ are reference points for tubes 1,2. Supplementary Movie 1 shows the entire time series in real time. (b) FeSO4induced RFP-labelled sperm cell (Sp) discharge. The image was captured in a single 250 ms exposure.Supplementary Movie 2shows a time series of ROS-induced sperm release. Scale bars (a,b), 50 μm. (c) Quantification of superoxide (generated by X/XO), H2O2and hydroxyl free radicals (generated by FeSO4-mediated Fenton reaction) induced pollen tube rupture. (d–f) Hydroxyl free radical scavengers suppressed ROS-induced tube rupture. Data=average±s.e.m. from at least triplicate from an analysis representative of three independent experiments;n=total number of pollen tubes examined. **P≤0.01 by Student’st-tests. Figure 4: ROS induce pollen tube rupture in vitro . ( a ) H 2 O 2 -induced tube rupture. The entire sample immediately prior to application of ROS (0 s) and when a majority of the pollen tubes has ruptured (3 m 40 s) (arrowheads point to cytoplasmic discharges) is shown in full. Magnified views of the first two rupturing pollen tubes (1, 2) are shown in between. * and Δ are reference points for tubes 1,2. Supplementary Movie 1 shows the entire time series in real time. ( b ) FeSO 4 induced RFP-labelled sperm cell (Sp) discharge. The image was captured in a single 250 ms exposure. Supplementary Movie 2 shows a time series of ROS-induced sperm release. Scale bars ( a , b ), 50 μm. ( c ) Quantification of superoxide (generated by X/XO), H 2 O 2 and hydroxyl free radicals (generated by FeSO 4 -mediated Fenton reaction) induced pollen tube rupture. ( d – f ) Hydroxyl free radical scavengers suppressed ROS-induced tube rupture. Data=average±s.e.m. from at least triplicate from an analysis representative of three independent experiments; n =total number of pollen tubes examined. ** P ≤0.01 by Student’s t -tests. Full size image ROS-induced pollen tube rupture is Ca 2+ -dependent To further probe the underlying process that lead to pollen tube rupture, we explored what potential targets ROS might use to trigger this response. Pollen tube growth is highly dependent on calcium [45] and ROS signalling is intimately linked to that of ion channel activation for example, that of Ca 2+ and K + (refs 39 , 43 , 44 ). Indeed, when pollen tubes were treated with ROS under different Ca 2+ conditions, tube rupture was suppressed in response to declining [Ca 2+ ] in the medium ( Fig. 5a ). Application of Ca 2+ channel blockers significantly reduced ROS-induced pollen tube rupture ( Fig. 5b,c ; Supplementary Fig. 7a,b ), whereas addition of even high concentrations of the K + channel inhibitor CsCl did not ( Fig. 5b ; Supplementary Fig. 7c,d ). Elongating pollen tubes are known to maintain a steep, tip-focused [Ca 2+ ] gradient [45] . Using Arabidopsis pollen tubes expressing a Ca 2+ reporter [46] , we observed abrupt increases in Ca 2+ in the distal cytoplasm within 1–2 min of ROS application ( Fig. 5c ; Supplementary Movies 3,4 ) and immediately preceding pollen tube rupture. Ca 2+ channel inhibitors effectively blocked Ca 2+ influx and inhibited rupture for at least half an hour in the presence of ROS, even when the apical Ca 2+ gradient was dissipated and growth became depolarized ( Fig. 5d ). In the ovules, progressively reducing [Ca 2+ ] in the pistil-feeding medium or adding EGTA to deplete endogenous Ca 2+ in excised pistils inhibited pollen tube rupture, inducing overgrowth ( Fig. 6 ). Taken together, these observations show that ROS-induced pollen tube rupture in vitro is dependent on Ca 2+ and Ca 2+ channel activation. They are also consistent with Ca 2+ being important for ROS-induced pollen tube rupture in the female gametophyte. Figure 5: ROS-induced pollen tube rupture is Ca 2+ dependent. ( a ) Effect of reducing [Ca 2+ ] on H 2 O 2 -induced pollen tube rupture. The excised pistils were pollinated and initially maintained in solidified medium containing 100 μM Ca 2+ to allow germination and tube growth prior to application of liquid medium containing 5 mM (standard) to 0 Ca 2+ . The level of tube rupture under 0 Ca 2+ treatment condition reflected the presence of minuscule amount of residual Ca 2+ contributed from the original growth medium. ( b ) Effects of inhibitors of Ca 2+ channel (LaCl 3 , GdCl 3 ) and K + channel (CsCl) on ROS-induced rupture. Pollen tube rupture was suppressed by LaCl 3 and GdCl 3 in a dose-dependent manner but was insensitive to CsCl and control reagents MgCl 2 and BaCl 2 [17] ( Supplementary Fig. 7a–d ). ( c , d ) Imaging intracellular Ca 2+ in a Ca 2+ -sensitive cameleon-expressing pollen tube during ROS (250 μM FeSO 4 )-induced rupture ( c ) and in the presence of 100 μM LaCl 3 ( d ). Heat maps reflect relative Ca 2+ levels. The 0 s images show high Ca 2+ at the tube apical region, typical of elongating pollen tubes [1] , [42] . * indicate the same position on the pollen tubes as reference points for growth during the observation period. LaCl 3 -treated tube continued growth during the treatment period (see distance between * and tip), slowed and developed apical swelling ( d ), but did not burst. Supplementary Movies 3 and 4 show the time series in ( c ). Scale bar, 10 μm. Data ( a , b )=average±s.e.m. from at least triplicate samples representative of three independent experiments; n =total number of pollen tubes examined. ** P ≤0.01 by Student’s t -tests. 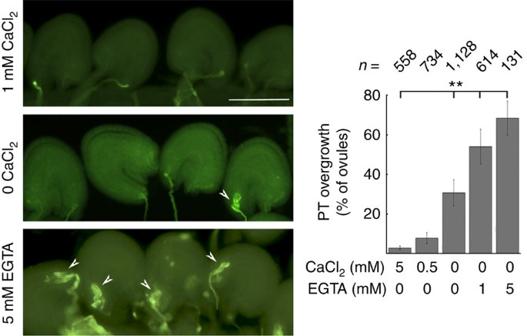Figure 6: Ca2+-dependent pollen tube rupture in the female gametophyte. Aniline blue-stained ovules show increasing level of pollen tube overgrowth in pollinated pistils fed with medium containing declining [Ca2+] or added EGTA (data=average±s.e.m. from triplicate samples (each with at least three pistils) representative of three independent examinations for individual treatment conditions;n=total number of ovules examined. **P≤0.01 by Student’st-tests. Scale bar, 100 μm. Full size image Figure 6: Ca 2+ -dependent pollen tube rupture in the female gametophyte. Aniline blue-stained ovules show increasing level of pollen tube overgrowth in pollinated pistils fed with medium containing declining [Ca 2+ ] or added EGTA (data=average±s.e.m. from triplicate samples (each with at least three pistils) representative of three independent examinations for individual treatment conditions; n =total number of ovules examined. ** P ≤0.01 by Student’s t -tests. Scale bar, 100 μm. Full size image LORELEI also regulates female gametophytic ROS To ascertain that a high ROS condition at the entrance to the female gametophyte is indeed a predominant condition for mediating pollen tube rupture in the female gametophye, we examined the ROS status in the ovules of a fer -like mutant lacking the glycosylphosphatidylinositol-anchored protein LRE [14] , [15] . We confirmed that pollen tube overgrowth in lre-5 (ref. 15 ) approximated the level observed in fer-4 and occurred at levels significantly higher than in wild-type ovules, similar to previously reported ( Supplementary Fig. 8 ). ROS staining showed that lre-5 ovules also showed significantly reduced levels of ROS around the filiform apparatus/synergid cell region relative to wild-type ovules ( Fig. 7 ). That two molecules commonly mediate a high ROS environment in the female gametophyte and loss of their functions induces similar pollen tube overgrowth defects provide strong support for the high ROS region at female gametopyte entrance as critically linked to its ability to induce rupture of a penetrating pollen tube. 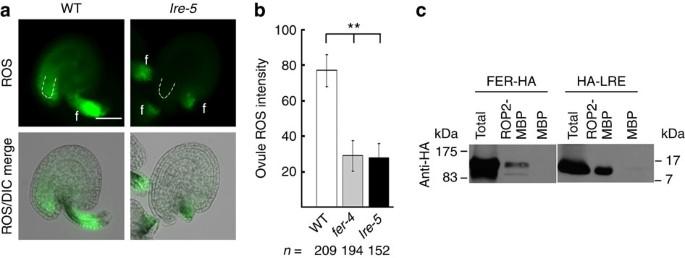Figure 7: LRE contributes to female gametophytic ROS and is a component of the FER-RAC/ROP signaling complex. (a) H2DCF-DA-stained wild-type andlre-5ovular ROS. f, funiculus, ROS occurred randomly, probably due to wound at the excision. (b) Quantification of filiform apparatus/synergid cell ROS in wild-type andlre-5ovules.Supplementary Fig. 8shows comparable levels offer-4andlre-5(refs14,15) female gametophytes displayed pollen tube overgrowth. Quantitative data are averages±s.e.m. of triplicate samplings (each with at least five pistils) from an analysis representative of three independent experiments; **, significant differences,P<0.01 by Student’st-test.n=total number of ovules examined. (c) ROP2-MBP pull down of FER-HA and HA-LRE. Immunoblot (upper) was stained by anti-HA antibodies to show the pulled down proteins. The FER pull-down result was similar to previously reported25and provides a comparison for LRE interaction with ROP2-MBP. The original scan and Ponceau-stained blot are shown inSupplementary Fig. 9. Figure 7: LRE contributes to female gametophytic ROS and is a component of the FER-RAC/ROP signaling complex. ( a ) H 2 DCF-DA-stained wild-type and lre-5 ovular ROS. f, funiculus, ROS occurred randomly, probably due to wound at the excision. ( b ) Quantification of filiform apparatus/synergid cell ROS in wild-type and lre-5 ovules. Supplementary Fig. 8 shows comparable levels of fer-4 and lre-5 (refs 14 , 15 ) female gametophytes displayed pollen tube overgrowth. Quantitative data are averages±s.e.m. of triplicate samplings (each with at least five pistils) from an analysis representative of three independent experiments; **, significant differences, P <0.01 by Student’s t -test. n =total number of ovules examined. ( c ) ROP2-MBP pull down of FER-HA and HA-LRE. Immunoblot (upper) was stained by anti-HA antibodies to show the pulled down proteins. The FER pull-down result was similar to previously reported [25] and provides a comparison for LRE interaction with ROP2-MBP. The original scan and Ponceau-stained blot are shown in Supplementary Fig. 9 . Full size image The similar ROS and pollen tube overgrowth phenotypes in fer and lre female gametophytes led to our considering that FER and LRE might act in a common pathway. We showed previously that FER interacts with ROPGEFs [25] , [31] and coexists with RAC/ROP GTPases in a tripartite signalling complex [25] . Using the same assay, we observed that LRE, like FER, was pulled down by ROP2 ( Fig. 7c ), thus implicating LRE as another component in the FER-RAC/ROP signalling complex working in concert with FER to impact female gametophytic ROS production. The discovery that FER-regulated ROS underlie reproductive success in Arabidopsis reveals a novel functional role for these ubiquitous regulatory molecules and provides mechanistic insight into a male and female interactive process that is crucial for flowering plant reproduction. ROS function in diverse ways [47] , [48] . For pollen tubes, ROS are required for their polarized growth [49] , [50] but they also mediate death as shown here ( Figs 3 , 4 , 5 , 6 ) and in self-incompatibility factor-treated pollen tubes [51] , suggesting different ROS-triggered processes could be involved. Plant cell growth requires constant balancing between cell wall extensibility to allow expansion and rigidity to provide integrity [52] and ROS are important for maintaining a balance between these two conditions [38] , [39] , [47] . A regulated ROS environment, for example via signalling through RAC/ROPs [25] , [53] , is important for cell growth such as in pollen tubes and root hairs. High levels of exogenously encountered ROS in the female gametophyte could over sever polysaccharides [54] and weakens the pollen tube wall, resulting in tube rupture, similar to enzyme treatment that disrupts cell wall properties [55] . The characteristics of ROS-induced pollen tube rupture described here provide insight on what might underlie the process. The Ca 2+ -dependent process in vitro and in the pistil suggests that Ca 2+ -signalled downstream events in the pollen tube could be involved. However, the almost instantaneous response upon exposure to ROS in vitro and penetration of the synergid cell in vivo would suggest that few pollen tube cytoplasmic signalling events are needed. The explosive nature of ROS-induced cytoplasmic and sperm discharge immediately following Ca 2+ channel opening ( Figs 4a,b and 5c ; Supplementary Movies 1–4 ) suggest possibly that a disrupted force equilibrium between turgor and cell wall strength underlies tube bursting. That medium osmolarity can modulate this process under normal and ROS-challenged growth conditions ( Supplementary Fig. 7e,f ) are consistent with this proposition. Although spatial constraint could not have been a factor in the ROS-induced catastrophic failure in pollen tube integrity in vitro , whether passage through a constricted environment [56] , like the filiform apparatus, contributes to the process remains to be determined. Increase in osmotic pressure has also been suggested as possibly underlying the species-specific ZmES4-induced pollen tube rupture that involves K + channel activation [17] , [57] . Whether ROS are involved in pre-conditioning the maize pollen tube for rupture is not known. Given that FER is conserved, ROS are ubiquitous, and pollen tubes from tobacco and lily also ruptured in response to ROS ( Supplementary Fig. 6h,i ), the FER-regulated pathway could be widespread to ensure reproductive success. It is intriguing to consider how an elongating pollen tube survives the high ROS environment at the filiform apparatus yet ruptures almost instantaneously upon penetrating the synergid. We suggest that Ca 2+ status across the synergid membrane at the filiform apparatus might underpin this process ( Fig. 8 ). A Ca 2+ -dependent pollen tube rupture process ( Figs 5 and 6 ) is consistent with a filiform apparatus [Ca 2+ ] on the extracellular side of the synergid cell membrane being below the threshold needed to induce rupture, preserving the integrity of a penetrating pollen tube. On the other hand, the synergid cytoplasmic Ca 2+ level could be high [58] , [59] , [60] and arrival of a pollen tube has been shown to increase the synergid [Ca 2+ ] in A. thaliana [60] . This could generate a [Ca 2+ ] high enough to trigger bursting of the invading tube. It could be envisaged that ROS encountered on the extracellular side of the synergid cell membrane could have weakened the pollen tube wall [54] , ‘priming’ it for rupture. Encountering the synergid cytoplasm, the already ROS-challenged tube would respond instantaneously to ROS-induced Ca 2+ -channel opening and abrupt water influx, leading to rupture. RAC/ROPs are known to regulate Ca 2+ fluxes [33] , [34] , loss of FER could have obliterated the rise of [Ca 2+ ] in the fer female gametophyte, thus preventing the Ca 2+ -mediated rupture of the penetrating pollen tube. On the other hand, as pollen tubes engage the FER relatives ANX1 and ANX2 to maintain its integrity throughout the tube growth process prior to entering the synergid cell, it cannot be discounted that the pollen tube itself may also be autogenously involved in ensuring its own rupture once inside the synergid [27] , [28] , [61] . Arrival at the female gametophyte and penetrating the synergid cell could have disengaged the function of ANX1 and ANX2, further lowering the ability of the penetrated pollen tube to resist rupture. 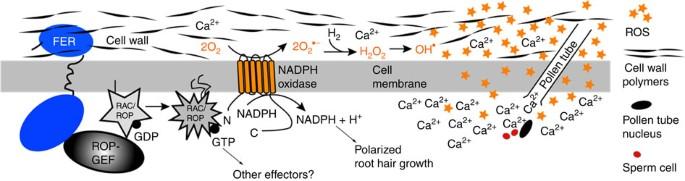Figure 8: RAC/ROPs and ROS as mediators of FER signaling. Both RAC/ROPs and ROS are known to regulate myriad biological processes, thus ideal for mediating the diverse functional roles of FER. NADPH oxidase is thus far the only downstream effector70demonstrated to mediate two major FER functional roles, polarized root hair growth and pollen tube rupture in the female gametophyte. Figure 8: RAC/ROPs and ROS as mediators of FER signaling. Both RAC/ROPs and ROS are known to regulate myriad biological processes, thus ideal for mediating the diverse functional roles of FER. NADPH oxidase is thus far the only downstream effector [70] demonstrated to mediate two major FER functional roles, polarized root hair growth and pollen tube rupture in the female gametophyte. Full size image It has been shown that pollen tubes from Arabidopsis lyrata and more distantly related Cardamine flexuosa do not burst in A. thaliana female gametophyte [24] . Whether FER participates in controlling cross-species incompatibility has not yet been investigated. It is possible to speculate that these cross-species pollen tubes might not be able to trigger a crucial event, for example, a Ca 2+ rise in the A. thaliana female gametophyte, as same-species pollen tubes do [60] , thus precluding a Ca 2+ level high enough to mediate ROS-induced bursting. The recent demonstration that a MYB-factor-controlled transcriptional program is important for sperm release in A. thaliana indicates certain pollen tube quality is necessary in this female–male interplay [19] , [21] . Differences in these qualities on the A. lyrata tube surface might preclude its bursting in the A. thaliana female gametophyte. It will be interesting to explore in the future whether FER directly contributes to the observed barrier of A. thaliana fertilization by incompatible cross-species pollen tubes. Understanding of how FER achieves its multiple functional roles is only emerging ( Fig. 8 ). The fact that FER also controls ROS-mediated polarized root hair growth [25] suggests these universal signalling molecules [39] , [47] , [48] could be common links for how FER mediates some of its diverse biological roles. The ROPGEF-RAC/ROP molecular switch serving as signal mediators for FER provides a perfect nexus where multiple signals can be integrated and diverse responses can be dispatched through a battery of distinct effectors [36] , [37] ( Fig. 8 ). Incorporating additional molecules, like LRE which functions almost as prominently as FER itself [14] , [15] , to mediate a specific response, in this case ROS-induced pollen tube rupture ( Fig. 7 ; Supplementary Fig. 8 ), might be a strategy whereby different FER functions can be executed depending on the presence of distinct partners. That the FER-controlled dual function in pollen tube–ovule interaction can be uncoupled ( Fig. 3c ) is also indicative of FER having the capacity to utilize distinct mechanisms to mediate different functions, even ones that are intimately linked. Plant growth conditions Arabidopsis thaliana was maintained at 22 °C in growth chambers [25] . Wild-type Col-0 and C24 were used as controls for fer-4 and srn , respectively. fer plants had pleiotropic phenotypes [12] , [13] , [25] , [29] , [30] , [31] , and were noticeably smaller and more stressed than wild type. Only the most robust fer plants were used in the analysis of their reproductive phenotype. lre-5 was as described [15] . pHTR10::HTR10-RFP-transformed Arabidopsis [62] was used as a marker line for sperm cells. Lat52:dtTomato transformed Arabidopsis was a gift from B. McClure (U. Missouri); it provided red fluorescence-labelled pollen tubes. Tobacco and lily were grown in greenhouses. Pollen tube growth assays Natural or hand-pollinated Arabidopsis pistils were used for in planta pollen tube growth analysis. The semi- in vivo pollen tube growth system [4] , [42] was used for in vitro tube growth analysis. A pistil-feeding system was developed to manipulate pistillate conditions and analysis of pollen tube growth in ovules. Each is described in the following sections. In planta analysis of pollen–ovule interaction Natural or hand-pollinated pistils from developmental stages 12–16 flowers [40] were used. Ovules in stage 14 and 15 flowers were at peak ovule receptivity [40] , [41] ( Supplementary Fig. 4a ). By stage 16, fertilization had occurred, sepals and petals had withered. Under our growth conditions, stages 13–15 spanned 36 h. For natural pollination, ovules from stages 14–15 flowers were used. For hand-pollination, stage 12b flowers based on female gametophyte development [41] (refer to as stage 12 in the text for simplicity) were emasculated and pollinated ~17 h later at the onset of stage 13. 20 h after pollination, pistils were fixed in FAA (10% formaldehyde, 5% acetic acid, 50% ethyl alcohol), softened in 1 M NaOH for 4 h, and stained with aniline blue to visualize pollen tubes [63] . Wild-type and pollen-specific Lat52::tdTomato [64] transformed pollen were used. Aniline blue-stained pollen tubes were visualized by epifluorescence (EX330-380/DM 400/BA420) in pistil squashes. tdTomato fluorescence protein-labelled pollen tubes were observed by epifluorescence (Ex546/10/DM 565 LP/Em 590 LP) after ovule excision. Analysis of pollen tube rupture in vitro The semi- in vivo pollen tube growth system [4] , [42] was used for in vitro Arabidopsis pollen tube growth and rupture studies because it supports robust in vitro growing pollen tubes and low levels of spontaneous rupture (see Fig. 4a,c and Supplementary Fig. 7e,f , see the standard cultures with 10% sucrose samples). Stage 12b flowers were emasculated and pollinated ~17 h later. Pollinated pistils were excised at the style/ovary junction and maintained in 3.5 cm petri dishes on solidified (0.7% agarose) germination medium [GM] [5 mM CaCl 2 , 5 mM KCl, 1.6 mM HBO 3 , 10% sucrose, pH7.5] [65] , unless modified as indicated in the text or figure legends. Pollen tubes emerged from the cut pistil after ~2–3 h. For mock and ROS treatments, standard medium or medium supplemented with various reagents, respectively were added around 1.5–2 h after pollen tubes had emerged from the cut pistils and observations were made 1 h after application of reagents except otherwise indicated. For treatments, all reagents were dissolved as suggested by manufacturers and diluted into 1 ml standard or modified GM for application to pollen tube culture. Tobacco and lily in vitro pollen tube growth conditions were as described [66] . Tobacco pollen tubes were cultured in 0.8 μM MgSO 4 .7 H 2 O, 1.6 μM H 3 BO 3 , 3 mM Ca(NO 3 ) 2 .4 H 2 O, 1 mM KNO 3 , 10 mM MES, pH 6.0, 8% sucrose, solidified with 0.7% agarose. Lily pollen tubes were cultured in 1.6 μM H 3 BO 3 , 1 mM KCl, 0.1 mM CaCl 2 , 15 mM MES, pH 5.5, 7% sucrose, solidified with 0.7% agarose. For ROS treatments: three different ROS reagents were used. First, H 2 O 2 (Fisher) was added to pollen tube cultures directly at the concentrations indicated. Second, 100 μM xanthine (Alfa Aesar)/0.2 U [X/XO] (CalBiochem) was added to generate superoxide. Third, FeSO 4 (Fisher) at the indicated concentration made in GM (adjusted to pH 6 to optimize the Fenton reaction without noticeably affecting pollen tube growth in control mock treatments) was added to pollen tube cultures to generate hydroxyl radicals via the Fenton reaction [43] , [44] , [67] . For ROS scavenger treatments: the hydroxyl radical scavengers sodium benzoate (Acros Organics), adenine (Sigma) and sodium salicylate (Sigma) and H 2 O 2 scavenger KI or sodium pyruvate [38] , [67] were applied in 1 ml of standard GM or modified with various reagents at the concentrations indicated in the figures for 10 min before application of 1 mM H 2 O 2 or 200 μM FeSO 4 . To determine the effect of Ca 2+ on ROS-induced pollen tube bursting, 1 ml of modified GM with 100 μM Ca 2+ was used in the solidified medium prior to ROS treatments. The low [Ca 2+ ] was needed to support pollen tube growth, which would not occur in Ca 2+ -free medium. For ROS treatment, H 2 O 2 (1 mM, or otherwise indicated) or FeSO 4 (200 μM) was applied in 1 ml of GM containing 0–5 mM (standard) Ca 2+ . Transformed Arabidopsis pollen tubes expressing the [Ca 2+ ] reporter yellow Cameleon YC3.6 (ref. 46 ) were used to monitor intracellular [Ca 2+ ] during ROS treatment (250 μM FeSO 4 ). To examine the involvement of Ca 2+ and K + channels in ROS-induced pollen tube bursting, Ca 2+ channel inhibitors GdCl 3 (MP Biomedicals, LLC) and LaCl 3 (ref. 43 ) (Santa Cruz Biotechnologies), and K + channel inhibitor CsCl [68] were added to pollen tube cultures 10 min prior to application of H 2 O 2 (1 mM) or FeSO 4 (250 μM) in GM. To examine the importance of osmoregulation for ROS-induced pollen tube bursting, 1 mM H 2 O 2 was applied in GM containing amounts of sucrose (5–15%) below or above, respectively, than in standard GM (10%). Excised pistil-feeding assays A pistil-feeding assay, whereby the pedicel of an excised pollinated pistil was immersed into medium ( Fig. 3a ) unsupplemented or supplemented with reagents, was developed to manipulate ovular conditions so as to examine factors that are important for pollen tube rupture. Pollen germination and tube growth in wild-type ( Fig. 3a ; Supplementary Fig. 5a ) and fer-4 ( Supplementary Fig. 5b ) pistils were not noticeably affected under mock treatment conditions. The outer three whorls of stage 12c flowers [40] , [41] were removed and their unpollinated pistils were excised from the base of the pedicel. The pedicel was planted into solidified (0.7% agarose) standard or modified GM in a sealed pipet tip. Chemicals used included DPI, an inhibitor of flavin-containing enzymes commonly used to determine NADPH oxidase dependence of ROS production, the superoxide scavengers tiron and CuCl 2 , the H 2 O 2 scavenger potassium iodide and sodium pyruvate and the hydroxyl radical scavenger sodium benzoate [38] , [39] , [67] ( Supplementary Fig. 3 ). Pistils were maintained for 6–8 h to allow reagent uptake, then pollinated by wild-type pollen, and kept for another 20 h in the same medium before processing for ovular ROS detection and aniline blue staining to visualize pollen tubes. The pistil-feeding assay was modified to assess Ca 2+ requirement on pollen tube rupture in the ovule because altering pistillate Ca 2+ conditions prior to pollination inhibited pollen germination and tube growth. Pistils were hand pollinated in planta to allow pollen germination and tube growth into the stigmatic papillae for 90 min prior to pistil excision and placed on modified GM with declining Ca 2+ or added EGTA. The excised pistils were laid sideways onto solidified GM ( Supplementary Fig. 7g ) for 20 h and then processed for observation. This allowed pistillate conditions to be altered without affecting pollen tube growth and targeting in the central transmitting tissues. Detection of ovular ROS Ovules were dissected from the pistil and immediately transferred to staining solutions at room temperature for whole mount observations. Staining and washes were carried out by absorbing used reagents by filter wedges and replenishing with new reagents or wash buffers. Each pistil was processed individually and routinely yielded ~20–30 undamaged ovules. H 2 DCF-DA [2′,7′-dichlorodihydrofluorescein diacetate] (Sigma), is highly sensitive to hydroxyl radicals among other oxygenated species [38] , [67] ; HPF (hydroxyphenyl fluorescein) (2-[6-(4′-hydroxy) phenoxy-3 H-xanthene-3-on-9-yl] benzoic acid (Cayman) is specific for hydroxyl radicals [38] , [67] , [69] . Ovules were immersed in 50 μM H 2 DCF-DA or 50 μM HPF in 50 μM CaCl 2 , 5 μM KCl, 10 mM MES, pH 6.15 at room temperature for 15 min. Samples were washed and observed immediately within a 5-min period. When used, DPI and various ROS scavengers described above were added under ROS-staining condition to concentrations described in the text. Where not indicated, data were from H 2 DCF-DA staining. We also tested Oxyburst green H 2 HFF-BSA (Invitrogen) that detects extracellular superoxide. It did not show signals internal to the micropyle, precluding its use in our studies. Imaging was carried out on a NIKON Eclipse E800 and captured by a SPOT CCD camera. H 2 DCF-DA- and HPF-detected ROS and JIM5-immunodetected pectin were observed by epifluorescence (Ex460-500, DM505, BA510-560). Data analysis and quantitative data presentation Unless otherwise indicated, data bars in histograms are the average±s.e.m. of at least three replicates from one representative experiment, which was repeated at least three times with comparable results. Experiments scoring ovule phenotypes examined at least three pistils (each of which yielded 20–30 undamaged ovules) per replicate. The average number of ovules and pollen tubes examined for the data shown are indicated in the figures as ( n ). Student’s t -test was used for statistical analysis. Differences with P ≤0.05 or P ≤0.01 (designated respectively by * and ** in figures) are considered significant. In most experiments, differences between control and experimental samples had P «0.01. Average signal intensity in regions of interest of identical areas at the filiform apparatus region (as shown in Supplementary Fig. 2 ) was quantified by ImageJ. Protein pull-down assay Escherichia coli produced ROP2-MBP and protoplast-expressed FER-HA and HA-LRE were used in protein pull-down assays as previously described [25] . Briefly, ROP2-MBP-bound amylose resin was used to pull-down FER-HA and HA-LRE expressed from the CaMV35S promoter in Arabidopsis protoplasts. 0.4% Triton X-100 soluble protoplast proteins were bound to the resin in 40 mM Tris-HCl (pH 7.5), 100 mM NaCl, 1 mM Na 2 -EDTA. After binding, the resin was washed five times in the same buffer. The bound proteins were eluted by direct resuspension and boiling in SDS–PAGE loading buffer and used for immunoblot analysis. Protein blots were stained by Ponceau (Sigma) to ensure comparable amounts of bait proteins were used. Anti-HA antibodies (Santa Cruz) were used to detect the pulled down FER-HA and HA-LRE. How to cite this article: Duan, Q. et al. Reactive oxygen species mediate pollen tube rupture to release sperm for fertilization in Arabidopsis . Nat. Commun. 5:3129 doi: 10.1038/ncomms4129 (2014).